Colloidal ribbons and rings from Janus magnetic rods Dipolar particles are fundamental building blocks in nature and technology, yet the effect of particle anisotropy is seldom explored. Here, we fabricate colloidal silica rods coated with a hemicylindrical magnetic layer to satisfy multiple criteria: nearly monodisperse, easily imaged and magnetic interaction that dominates over gravity. We confirm long-predicted features of dipolar assembly and stress the microstructural variety brought about by shape and constituent anisotropy, especially by extrapolating knowledge learned from literal molecules. In this colloidal system, we describe analogies to liquid crystalline deformations with bend, splay and twist; an analogy to cis / trans isomerism in organic molecules, which in our system can be controllably and reversibly switched; and a field-switching methodology to direct single ribbons into not only single but also multiple rings that can subsequently undergo hierarchical self-assembly. We highlight subtle material issues of control and design rules for reconfigurable dipolar materials with building blocks of complex shape. Spontaneous assembly of objects with permanent dipoles governs association on many length scales in natural and technologically relevant systems [1] : at the molecular level, polar molecules such as water and chloroform; at the nanoparticle scale [2] , [3] , ferrofluids [4] and magnetosomes in magnetotactic bacteria [5] , [6] ; and at human scales, various magnetic tools and toys. To date, experimental studies have mainly focused on materials in which electric or magnetic dipoles exist solely due to the presence of externally applied fields [7] , [8] , [9] , [10] . Here, we introduce a new system composed of magnetic Janus rods that possess permanent dipoles and, referring to their association as dipolar assembly, explore their assembly into unique and interesting structures with analogies to liquid crystalline materials and organic molecules. Experiments lag behind extensive theory and simulation of dipolar assembly, even for spheres [11] , [12] , [13] , [14] , [15] , [16] , [17] , [18] , [19] . On the experimental side, structures of ferromagnetic nanoparticles were inspected by cryogenic electron microscopy [20] , [21] , but all dynamics were missing owing to the sample preparation. Granular particles can be made monodisperse and studied in real time, but their large size means that gravity dominates over the intrinsic dipolar interaction, limiting the system to two dimensions [22] , [23] , [24] . Here, we consider dipolar particles of intermediate size: ones that are small enough that the dipolar interaction can overwhelm gravity, yet large enough to visualize optically in real time, and that possess uniform magnetic properties. Although some particles of this kind were known from earlier work by others, previous emphasis was on their assembly or dynamics in the presence of external magnetic field [25] , [26] , [27] , [28] , [29] , [30] , [31] . Here, taking advantage of rapid progress in the synthesis of anisotropic colloids [32] , [33] , [34] , [35] , [36] , [37] , we go beyond this to delve into the role of shape and constituent anisotropy. Beyond validating and testing the generality of theoretical and in silico predictions regarding dipolar assembly, these findings shed new light on the design of reconfigurable materials [38] in which large structural transitions can arise from small changes in field strength [39] . Synthesis of magnetic Janus rods To implement the goal of monodisperse size and homogeneous magnetic response, we take the approach of directionally depositing thin magnetic coatings onto monodisperse colloids [27] , [28] , [29] , [40] , [41] . To realize shape anisotropy, we first prepare silica rods that are 2.4±0.1 μm long and 0.81±0.04 μm wide (that is, an aspect ratio of 3), using a known method [42] . They are further coated on one hemicylinder with a nickel layer 9.8 nm thick. The strength of the dipole moment can be precisely controlled by the rod dimension and coating thickness. The Ni layer is further protected by a 15 nm layer of SiO 2 . This layer makes the particle surface chemically isotropic, such that surface-induced interaction anisotropy does not come into play; meanwhile, it raises the particles’ surface charge (zeta potential of −43±4 mV). We study magnetic assembly in deionized (DI) water, where the strong electrostatic repulsion prevents the particles from uncontrolled aggregation or adsorption onto the sample chamber from van der Waals attraction or gravitational pinning. The parameters employed in the current study minimize unwanted aggregation while ensuring dominance of magnetic energy (~10 3 k B T ) (balanced by electrostatic energy) over thermal energy and gravitational energy (~ k B T ). Supplementary Figs S1,S2 show examples of the geometrical uniformity of the rods before and after coating, respectively. Ribbon formation We found a simple method to remedy the fact that as-synthesized particles possess magnetic moments of uncontrolled orientation with respect to their long axis. When subjected to a magnetic field much larger than their coercive field, individual rods align their long axis perpendicular to the field and subsequently stack into ribbons parallel to the field ( Supplementary Fig. S3 ), regardless of their initial magnetization direction. Turning off the field at this point does not change the acquired magnetization direction. The findings were the same regardless of coating thickness or rod aspect ratio, when these parameters were varied in control experiments. The origin of the observed magnetization direction along the short axis is not understood, but it is convenient in constructing building blocks for the present experiments because it favours rods to arrange side-by-side, a phenomenon that we exploit in the assembly described below. After the magnetic field is turned off, stray field from ambient objects and the earth’s magnetic field are compensated using a homebuilt triaxial magnetic setup (see Methods and Supplementary Fig. S4 ), resulting in near-zero magnetic field (±0.05 G). The ribbons display flexibility, yet retain their integrity owing to remnant moments of the nickel coating. Ribbons point in random directions and form a beautiful labyrinthian pattern ( Fig. 1a ), confirming vividly a theoretical prediction made long ago [13] , [14] . 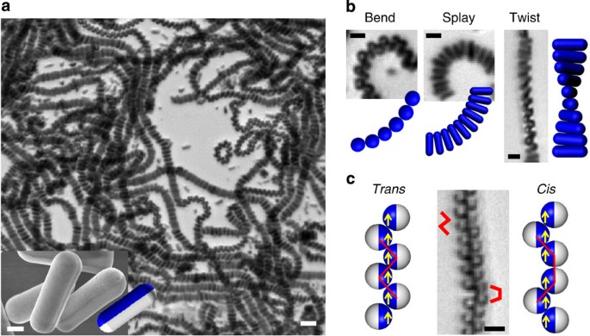Figure 1: Ribbons of dipolar Janus rods at zero magnetic field. (a) Representative optical image of a concentrated suspension of the dipolar Janus rods. The image includes some solitary uncoated particles, which do not interfere with the dipolar assembly. Scale bar, 5 μm. Inset: representative scanning electron microscopy image of individual rods with schematic representation, in which blue represents the nickel-coated side and white the bare silica side. Scale bar, 0.5 μm. (b) Liquid-crystal-like deformation modes of a colloidal ribbon, images accompanied by schematic illustrations. For clarity, the Janus feature is not illustrated. Scale bar, 2 μm. (c) End-on view of a ribbon in a small vertical field (1.6 G), accompanied by schematic illustrations highlighting thetransandcisbonds. Yellow arrows denote the dipole moment of each rod. Red lines highlighttransandcisbonds. Scale bar, 2 μm. Figure 1: Ribbons of dipolar Janus rods at zero magnetic field. ( a ) Representative optical image of a concentrated suspension of the dipolar Janus rods. The image includes some solitary uncoated particles, which do not interfere with the dipolar assembly. Scale bar, 5 μm. Inset: representative scanning electron microscopy image of individual rods with schematic representation, in which blue represents the nickel-coated side and white the bare silica side. Scale bar, 0.5 μm. ( b ) Liquid-crystal-like deformation modes of a colloidal ribbon, images accompanied by schematic illustrations. For clarity, the Janus feature is not illustrated. Scale bar, 2 μm. ( c ) End-on view of a ribbon in a small vertical field (1.6 G), accompanied by schematic illustrations highlighting the trans and cis bonds. Yellow arrows denote the dipole moment of each rod. Red lines highlight trans and cis bonds. Scale bar, 2 μm. Full size image Analogies to molecular assembly Moving from macroscopic patterns to microstructural features, we note two analogies to molecular assembly: deformations akin to those in liquid crystals and neighbour–neighbour arrangement akin to cis / trans conformations of the double bond in organic molecules. The former results from the elongated shape and the latter from the Janus feature. Together, they add richness and controllability to the dipolar self-assembly process. Specifically, close inspection of Fig. 1a reveals three types of deformation on the ribbon: bend, splay and twist ( Fig. 1b ), reminiscent of the classic deformation modes of liquid crystals [43] . Bend, which refers to deformations in a plane looking into the rods such that their cross-section is circular, is energetically least costly. Splay, which refers to deformation in the plane of the rods, is more energetically costly. Even more costly, pure twist is observed, but only under special conditions (see Methods). The effect of constituent (Janus) anisotropy is also manifested in the ribbon geometry. Consider a view looking end-on into these ribbons such that the cross-section of a rod is a circle ( Fig. 1c ). As the magnetic material is distributed on just one hemicircle (hemicylindrical in three dimensions), the dipole moment is shifted away from the geometrical centre towards the coated side [44] . This shift gives rise to two ways in which the rods may line up. The most stable configuration is a zig–zag chain in which particles alternately face one another, which we call the trans configuration in analogy to a carbon–carbon double bond. Another possibility observed is the cis configuration, in which the magnetic sides of two neighbouring rods face the same direction. This configuration is higher in energy, Δ E (estimated Δ E ≈1.3 × 10 3 k B T per pair, see Supplementary Fig. S5 and Supplementary Note 1 ), because the dipole separation between neighbouring particles is larger. It is also metastable, as the conversion from a cis to trans configuration requires 180° rotation of half a chain with respect to the other half, which involves a highly twisted intermediate state. Hence, both the kinetics and thermodynamics of these trans/cis bonds are similar to their molecular analogue in carbon double bonds. From time-lapse movies of the ribbon formation process, we find that particles always adopt the trans configuration when they add individually to the end of a ribbon, but that when two ribbons link ( Supplementary Movie 1 ), there is a chance to be trapped in a cis configuration. Therefore, statistically each ribbon possesses both cis and trans bonds, the latter being more abundant. Note ( Fig. 1c , middle panel) that a cis bond introduces a kink in an otherwise-straight pure trans chain. The interesting consequences are discussed below. Dynamics of ring formation: buckling and splitting into daughter rings Now we turn to dilute conditions in which ribbons do not interact. Static energy calculation of dipolar spheres at zero field show that rings represent the minimum energy configuration [16] . Attraction between ends should always dominate bending energy, the latter resulting from misalignment between neighbouring dipoles in a bent chain. A lingering question is what pathway leads to this energy minimum. Conventional simulation starts from an isotropic distribution of particles, a situation relevant to the nature of phase transition and associated aggregation kinetics in dipolar fluid [45] ; but the alternative approach of watching relaxation from an existing chain is interesting from a materials point of view. It is predicted that to reach a ring state, a large kinetic barrier of bending, before ends come sufficiently close to attract, can prohibit this transformation in zero field [46] . However, we find that by switching the field direction, ribbons can be directed into cyclic structures. The ribbon tries to follow the reversal of the field, but not instantaneously owing to viscous drag, which causes the ribbon to buckle [47] , [48] in different ways and ultimately leads to different fates. 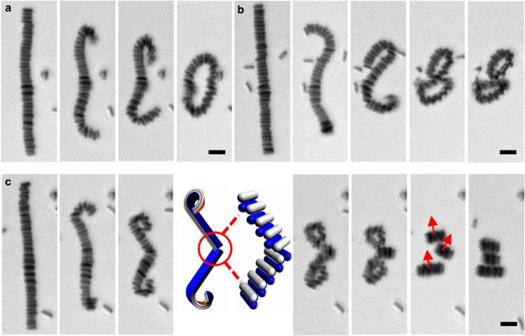Figure 2: How cyclic structures of dipolar Janus rods form from linear ribbons when reversing the field. (a) In this example, a single ring forms from a C-shaped intermediate. From left to right:t=0, 1.33, 1.86 and 2.64 s. (b) In this example, a ribbon splits into two rings via S-shaped and figure-8-shaped intermediates. From left to right:t=0, 3.08, 4.16, 4.86 and 5.73 s. (c) In this example, a ribbon splits into three rings. From left to right:t=0, 2.05, 2.51, 2.86. 3.05, 4.62 and 13.9 s. Included is a schematic illustration of the intermediate state as well as an enlarged view of the discontinuity. The red arrows indicate the collective dipole of the daughter rings. Scale bar, 4 μm. Figure 2 shows three outcomes from repeated experiments on the same ribbon when reversing the field. Ends always follow the field reversal faster than the main body. If they curve in the same direction, further relaxation results in a completed loop ( Fig. 2a , Supplementary Movie 2 ). If they curve in opposite directions, the ends cannot meet, so the ribbon simply reverses direction via an S-shaped intermediate. But often, the S-shaped intermediate collapses transiently into a figure-8 shape ( Fig. 2b , Supplementary Movie 3 ), which subsequently splits in the middle to form two separate rings. Further complexity arises when the magnetic field reverses direction rapidly. Under these conditions, even if the ends curve in the same direction, the splayed middle section can suddenly develop a singularity that absorbs the curvature ( Fig. 2c ). The splay deformation is not only one of higher energy, but also more susceptible to failure by undergoing twist around a single bond, as shown in the schematic representations in Fig. 2c . In this particular case, the ribbon finally breaks into three pieces, each of which forms an individual small ring. As analysed below, such rings have a collective dipole perpendicular to their contour, causing them to align with the field and undergo hierarchical assembly into stacks (see Supplementary Movie 4 ). If this could be scaled up, it suggests the possibility of forming tubular structures spontaneously from single ribbons [49] . The Supplementary Movies 2–5 offer more examples of how ring formation depends on pathway. In addition to the rate of field reversal, we find that the ring formation dynamics also depend on many other factors, especially the initial orientation relative to the sample substrate and the presence of cis bonds, revealing the richness of these phenomena. Figure 2: How cyclic structures of dipolar Janus rods form from linear ribbons when reversing the field. ( a ) In this example, a single ring forms from a C-shaped intermediate. From left to right: t =0, 1.33, 1.86 and 2.64 s. ( b ) In this example, a ribbon splits into two rings via S-shaped and figure-8-shaped intermediates. From left to right: t =0, 3.08, 4.16, 4.86 and 5.73 s. ( c ) In this example, a ribbon splits into three rings. From left to right: t =0, 2.05, 2.51, 2.86. 3.05, 4.62 and 13.9 s. Included is a schematic illustration of the intermediate state as well as an enlarged view of the discontinuity. The red arrows indicate the collective dipole of the daughter rings. Scale bar, 4 μm. Full size image Non-circular complex rings After forming cyclic configurations, we cancel the field such that rings adopt configurations without interference from external field. Under this circumstance, we always observe rings to lie parallel to the substrate owing to gravity, such that their cross-sectional shapes as well as cis/trans configurations can be visualized ( Fig. 3 ). Rings composed only of trans configurations assume the circular shape long known to hold for dipolar spheres [11] ( Fig. 3a-1 ). However, cis bonds introduce kinks that subsequently determine the ring shape. Rings with a single cis bond assume a raindrop shape ( Fig. 3a-2 ). A compelling illustration is Supplementary Movie 6 , showing the dynamic transition from circular to raindrop shape via the addition of a single cis bond. Rings with two equally spaced cis bonds are football-shaped ( Fig. 3a-3 ). Three equally spaced cis bonds define three vertices of a triangle ( Fig. 3a-4 ). The same trend extends to squares ( Fig. 3a-6 ) and even larger polygons. In addition to this dependence on the number of cis bonds, obviously their shapes also depend on the distance between them (compare Fig. 3a-4 ). In the future, it may be desirable to find ways to precisely control the number and positions of cis bonds, permitting one to engineer polyhedral shapes via dipolar self-assembly. 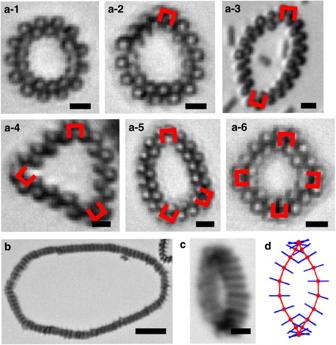Figure 3: Optical images of dilute cyclic structures formed from dipolar Janus rods at zero field. Panelashows an inventory of ring shape with all-bend deformations: An all-transconfigurations produce circular rings (a-1). A singlecisbond (highlighted by the red symbol) produces a raindrop shape (a-2). Two equally spacedcisbonds shape a football (a-3). Equilateral (a-4) and isosceles (a-5) triangles result from threecisbonds. From four equally spacedcisbonds, a square results (a-6). Scale bar, 2 μm. (b) A large ring formed solely by splay deformation. Scale bar, 10 μm. (c) Ring with mixed deformation in a small (1.5 G) horizontal field, with a schematic representation (d) generated by following Euler coordinates51. Scale bar, 2 μm. Figure 3: Optical images of dilute cyclic structures formed from dipolar Janus rods at zero field. Panel a shows an inventory of ring shape with all-bend deformations: An all- trans configurations produce circular rings ( a-1 ). A single cis bond (highlighted by the red symbol) produces a raindrop shape ( a-2 ). Two equally spaced cis bonds shape a football ( a-3 ). Equilateral ( a-4 ) and isosceles ( a-5 ) triangles result from three cis bonds. From four equally spaced cis bonds, a square results ( a-6 ). Scale bar, 2 μm. ( b ) A large ring formed solely by splay deformation. Scale bar, 10 μm. ( c ) Ring with mixed deformation in a small (1.5 G) horizontal field, with a schematic representation ( d ) generated by following Euler coordinates [51] . Scale bar, 2 μm. Full size image Occasionally, Möbius strips [50] are observed, but they are only transient owing to the large twisting energy. Rings with pure splay deformation are also observed ( Fig. 3b ), provided that repeating units within a ribbon are sufficiently many. Field response A converse question to how rings form is: what happens to cyclic structures when a small magnetic field is applied? Ultimately, they must break into ribbons that align with the field; but understanding the dynamic route is of interest. We observe beautiful pathways from the ring to ribbon states, and in contrast to the many ways that rings can form, their rupture kinetics are deterministic, robust and general (see Supplementary Movie 7 ). 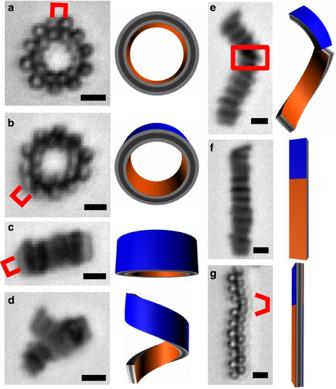Figure 4: How a ring of dipolar Janus rods deforms and breaks in response to a small field. Each optical image is accompanied by a schematic illustration where dark grey represents the line of magnetic dipoles holding the ring together. Blue and orange are guides to the eye to distinguish outer and inner sides of the original ribbon ring. In going from 0.2 to 2.1 G, the ring first rotates in the image plane from (a,b), then out of plane from (b,c). Increasing further to 2.7 G, rupture dynamics initiates from (d), leaving a large twist on the ribbon that releases by rotating the top half with respect to the bottom half in (e); the flipped bond is highlighted. Finally, a linear ribbon results (f), which is forced to stand up in (g) by applying a 10 G field at 20 Hz perpendicular to the image, showing the newborncisbond. Scale bar, 2 μm. Figure 4 shows snapshots of a ring containing one cis bond, responding to a small vertical field in the image plane. In this example, the ring first rotates in the image plane, placing the cis bond on one side ( Fig. 4b ). It then stands up on the substrate, perpendicular to the external field, such that in the image one observes a side view of the ring ( Fig. 4c ). Standing-up behaviour signifies that the ring acquires a collective dipole moment perpendicular to itself. Figure 4: How a ring of dipolar Janus rods deforms and breaks in response to a small field. Each optical image is accompanied by a schematic illustration where dark grey represents the line of magnetic dipoles holding the ring together. Blue and orange are guides to the eye to distinguish outer and inner sides of the original ribbon ring. In going from 0.2 to 2.1 G, the ring first rotates in the image plane from ( a , b ), then out of plane from ( b , c ). Increasing further to 2.7 G, rupture dynamics initiates from ( d ), leaving a large twist on the ribbon that releases by rotating the top half with respect to the bottom half in ( e ); the flipped bond is highlighted. Finally, a linear ribbon results ( f ), which is forced to stand up in ( g ) by applying a 10 G field at 20 Hz perpendicular to the image, showing the newborn cis bond. Scale bar, 2 μm. Full size image To our knowledge, it is the first observation of this long-predicted behavior [11] , which arises because the magnetic attraction dominates over gravity at the colloidal scale, allowing the ring structure to rotate in three dimensions. For spheres, the mechanism was predicted to be a simultaneous rotation in the external field direction of all spheres’ dipoles, adding up to an overall moment perpendicular to the ring. In these experiments, the rods have the same tendency; however, they cannot do so without hitting one another owing to their geometric shape and the steric constraint of tracing a circle. This excites collective deformations of the ring contour, visible in the side view for a larger ring ( Fig. 3c ). Distortion on a circle formed by a ribbon has been predicted to simultaneously excite three deformation modes [51] : not only bend, but also splay and twist must come into play. Figure 3d shows that the observed conformation is consistent with a hypothetical sinusoidal variation of rod angle moving along the ring’s contour (see Supplementary Note 2 ), although detailed energy calculation awaits further study. Spiral rupture Rings break predictably at their weakest spots, the cis bonds, when the magnetic field exceeds a limit dependent on the specific ring size and configuration, such as the number and position of the cis bonds ( Fig. 4d ). The qualitative feature of breakage dynamics is robustly observed for all rings without defects: ring breakage generates two ends that go in opposite directions, giving a spiral breakage mode [23] . The middle part of the ribbon is then left in an awkward configuration: it contains a large twist in addition to bend and splay, which is the highest-energy deformation. To release twist from that state, one half of the ribbon must rotate with respect to the other half, around the bond indicated by the red box in Fig. 4e . This converts a trans bond into a cis bond, as shown by the side view of the resultant ribbon ( Fig. 4g ). The reverse transformation from cis to trans bond can also take place ( Supplementary Fig. S6 ). It was shown recently that mechanical force can switch the configuration of double bonds in organic molecules [52] ; here we see a colloidal analogue of this interesting phenomenon. Importantly, this allows some control over the number and position of cis bonds on a ring. Transient helices Intriguing collective dynamics arise for strongly coupled rings (see Supplementary Movie 8 ). 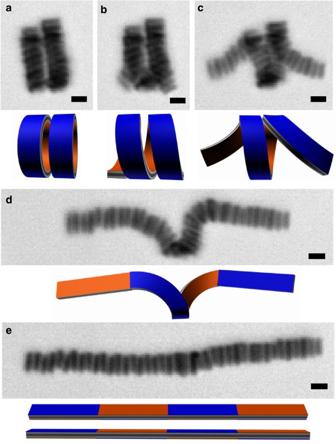Figure 5: How two stacked rings collectively evolve into one single ribbon. In this example, the field increases from 1.3 to 1.8 G in the horizontal direction, in a time series from (a–e) 0, 0.58, 0.94, 1.82 and 3.03 s, respectively. Schematic depictions of the ribbon state accompany each structure. Scale bar, 2 μm. The colour usage is the same asFig. 4. Figure 5a shows two standing-up rings in a small horizontal field. They stand side-by-side because of their collective dipole moments; their similar size leads to similar threshold field for rupture. As shown in Fig. 5b , at the time of breakage the top part of the left ribbon moves to the right and its bottom part moves to the left, or vice versa , and the same is true for the right ribbon. Hence, the top end of the left ribbon meets the bottom end of the right ribbon, connecting the two ribbons into one. This gives a transient helical structure, as depicted in a schematic illustration ( Fig. 5b ). Although it is possible to produce helical colloidal springs and related structures as a provocative proof of concept ( Supplementary Fig. S7 ), chemical advances would be needed to render them permanent. Figure 5: How two stacked rings collectively evolve into one single ribbon. In this example, the field increases from 1.3 to 1.8 G in the horizontal direction, in a time series from ( a – e ) 0, 0.58, 0.94, 1.82 and 3.03 s, respectively. Schematic depictions of the ribbon state accompany each structure. Scale bar, 2 μm. The colour usage is the same as Fig. 4 . Full size image By synthesizing monodisperse Janus magnetic particles, we have created a new model system in which to study self-assembly based on permanent dipoles. These building blocks, anisotropic in both shape and chemical constituents, enable one to test some of the classical predictions from extensive theory and simulation [11] , [12] , [13] , [14] , [15] , [16] , [17] , [18] , [19] , although to do so is not the main point of this study. The microscopic size of our rods allows direct visualization of dynamic pathways of the resulting dipolar rings in response to external fields. Some of these dynamic features were previously observed in granular particles of much larger size, but in granular systems gravity restricts particles to two dimensions. The present system allows rotation of individual building blocks as well as their assemblies in three-dimensional space. We therefore observe inherent three-dimensional dynamic features of these dipolar structures, uninfluenced by the much weaker gravity. Looking to the future, it is evident that enhanced image quality and genuine three-dimensional information could be obtained by implementing fluorescent-core silica rods coupled with confocal microscopy, which we have not pursued here. Extensive earlier theoretical interest about dipolar particles dwelt on their equilibrium configuration and resulting phase diagrams starting from the isotropic state [17] . By contrast, here we stress their microstructural variety. Borrowing a language developed to describe molecules, we show that colloidal-scale cis/trans isomerism gives ribbons with kinks, which subsequently form rings of non-circular contour with bend, splay and twist deformations akin to liquid crystals. Above a threshold external field, they interconvert via well-defined pathways with rupture initiated at spatially localized kinks. Our observations provide design rules for reconfigurable dipolar materials with building blocks of complex shape. Our observations were qualitatively the same when, in addition to Janus magnetic rods of aspect ratio of 3 reported in detail above, we also tested rods with aspect ratios of 2 and 4, as well as Ni-coating thicknesses varied from 10 to 20 nm, above which irreversible aggregation occurs. Extensions of these ideas to other particle shapes [53] are evident. For example, for cubic particles [26] , there is a tendency for three cubes to form a defined 90° kink rather than uniform bending, hence the ring might be inherently rectangular. In the future, it should also be possible to design multiple magnetic patches on a single colloid [26] , [37] . Such particles might under some situations behave as a gross dipole, under other situations interact through different patches separately, leading to interesting control possibilities. It is intriguing that the seemingly simpler system of magnetic Janus spheres did not display such rich phenomena. For the choice of materials studied here, Janus magnetic spheres collapse into hexagonal sheets in which all particles face their magnetic side in the same direction of surface normal ( Supplementary Movie 9 ), in zero magnetic field. These sheets align with their surface normal perpendicular to the external field [54] , prohibiting formation of circular structures. The generality of this observation is unclear, as it might be related to the way the actual magnetic material is distributed on a Janus sphere [40] , as well as to the specific magnetization direction and strength, but it does present the example of a system in which magnetic Janus spheres do not necessarily assemble into rings. For Janus rods, this hexagonal packing is simply not available, for geometric reasons. Hence, the unique combination of elongated shape and Janus character of these colloids is not merely a convenient choice, but an essential one to realize the complex ring conformations and diverse dynamics reported here. However, the assembly of Janus magnetic spheres under time-dependent magnetic fields does present other interesting issues involving the selection of structures that can tolerate synchronized motion. [55] Looking to the future, we note that the surface-coating methods employed here lend themselves to such studies of dipolar particles in facile ways. First, they allow realization of any particle shape provided that the starting monodisperse material is available. Second, variations of the coating thickness allow precise control of the dipole strength. Third, variations of the shape anisotropy, as in our case, or incorporation of special magnetic films [41] , allow precise control of the dipole orientation. To conclude, this paper demonstrates a self-assembly paradigm for creating field-responsive colloidal assemblies that are dynamically reconfigurable and possess interesting instability modes and rich kinetic pathways. Implemented here for magnetic rods using methods readily extendable to other particle shapes, dipolar colloids with constituent (Janus) and shape anisotropy are shown to display dipolar assembly that shares some of the long-predicted features of dipolar spheres, yet differ from what has been predicted for spheres. There are fundamental consequences from loss of symmetry on the single-particle level. This causes, on the assembly level, inhomogeneous distributions of stress arising from constituent anisotropy and new deformation modes arising from anisotropic shape, resulting in major new pathways of rational design and control. Particle synthesis The silica rods are synthesized by slight modification of a known procedure [42] . We introduced a filtration step to achieve more monodisperse emulsion droplets for the nucleation process, which leads to highly monodisperse silica rods. The initial synthesis results in rods 1.9±0.2 μm in length and 0.31±0.05 μm in diameter. Seeded Stöber processes are used to grow additional layers of silica. After 13 additions of water and tetraethyl orthosilicate, the rods are 2.4±0.1 μm in length and 0.81±0.04 μm in diameter as manually measured from scanning electron microscopy images. Rods of aspect ratios of 2 and 4 are synthesized in a similar way. To produce magnetic coatings, the rods are then dried and resuspended in DI water at 1% weight concentration. A 20 μl suspension is spread onto a half glass slide (1.0 × 1.5 inch) pretreated with Piranha solution, and dried quickly to form a submonolayer of rods lying parallel to the glass. The drying edge of the glass contains multilayers with ill-defined orientation; it is covered with a glass slide during the metal deposition and removed later. A 9.8 nm nickel coating followed by a 15 nm SiO 2 coating is then vertically deposited using electron-beam deposition. In control experiments, we also tested Ni-coating thicknesses from 10 to 20 nm. A control glass slide without particles is coated simultaneously and used to measure the film thickness by ellipsometry (J.A. Woollam VASE ellipsometer). The monolayer is washed thoroughly with DI water and isopropyl alcohol, and then sonicated in 15 ml DI water to collect the particles. In DI water, the particles have a zeta potential of −43±4 mV (Malvern Zetasizer Nano). Scanning electron microscopy images are taken in a Hitachi S4800 electron microscope with particles without SiO 2 layer to improve contrast. Setup A spatially homogeneous magnetic field with controllable x , y and z components is generated by three orthogonal pairs of solenoids (Science Source #14835 with iron cores, and custom-designed coils from Teachspin), controlled by three power supplies (Kepco 100-4D). We install a Gaussmeter (Alpha Lab, Model VGM) from the side (see Supplementary Fig. 4 for setup image) to monitor the field at the centre during all experiments. The conversion factor of the reading of the monitoring Gaussmeter to the actual field under which assembly takes place is calibrated with a second Gaussmeter placed at the focus of the objective. During the experiment, zero magnetic field is defined as the field strength when ribbons show random orientations. Movies are taken in a home-built microscope using an LED light source (Thorlabs MCWHL2), a × 50 long-working-distance objective (Mitutoyo, Numerical aperture=0.55) and a complementary metal–oxide–semiconductor camera (Edmund Optics 5012M GigE). Assembly protocol A 400 μl suspension (~10 −2 mg ml −1 ) of the Janus rods is introduced into the imaging chamber (Lab-Tek II chambered cover glass). The particles sediment but negative charges on the silica particles prevent adsorption to the chamber walls as well as irreversible clustering of particles. A static field with strength up to 200 G is applied overnight to assemble the rods into ribbons. Then, the field strength in each direction is carefully tuned by the power supplies to ensure no preferential alignment of the ribbons; this, we defined as zero field. To form rings, first we cancel the field in two directions, then reverse the field direction along the remaining axis. After rings form, we relax back to zero field in all directions to observe the zero-field configuration. For the breakage dynamics, we slowly increase the field strength in one axis. To force the ribbon to stand up (in order to check the trans/cis configuration), we apply an additional alternating field of 10 G at 20 Hz in the z direction, perpendicular to the image. To observe twisting modes, a precessing field [55] of 50 G at 20 Hz and precession angle of 20° is applied with precession axis vertical in the image plane. Ribbons align parallel to the precession axis of the external field and rotate around their long axis. Meanwhile, they show significant twisting owing to uneven distribution of torque. How to cite this article: Yan, J. et al . Colloidal ribbons and rings from Janus magnetic rods. Nat. Commun. 4:1516 doi: 10.1038/ncomms2520 (2013).